The RB family is required for the self-renewal and survival of human embryonic stem cells The mechanisms ensuring the long-term self-renewal of human embryonic stem cells are still only partly understood, limiting their use in cellular therapies. Here we found that increased activity of the RB cell cycle inhibitor in human embryonic stem cells induces cell cycle arrest, differentiation and cell death. Conversely, inactivation of the entire RB family (RB, p107 and p130) in human embryonic stem cells triggers G2/M arrest and cell death through functional activation of the p53 pathway and the cell cycle inhibitor p21. Differences in E2F target gene activation upon loss of RB family function between human embryonic stem cells, mouse embryonic stem cells and human fibroblasts underscore key differences in the cell cycle regulatory networks of human embryonic stem cells. Finally, loss of RB family function promotes genomic instability in both human and mouse embryonic stem cells, uncoupling cell cycle defects from chromosomal instability. These experiments indicate that a homeostatic level of RB activity is essential for the self-renewal and the survival of human embryonic stem cells. Embryonic stem cells (ESCs) and induced pluripotent stem cells have an unlimited proliferative and self-renewal potential but also maintain the ability to differentiate into a wide array of cell types, making them ideal candidates for use in targeted cellular therapies [1] . However, the tumorigenic potential of human ESCs (hESCs) and induced pluripotent stem cells remains a concern, and directing their differentiation into specific cell types is challenging [2] . Overall, the mechanisms regulating the basic properties of hESCs are still not well understood, hampering the development of novel therapeutic strategies. ESCs have a shorter G1 phase of the cell cycle as compared with most other cell types, including adult stem cells, which are often quiescent. Cell cycle arrest in G1 is thought to be permissive for differentiation in ESCs, whereas it is associated with maintenance of stemness in adult stem cells [3] , [4] , [5] . Functional differences in the cell cycle machinery of hESCs in comparison to adult stem cells and ESCs and epiblast stem cells (EpiSCs) from other species are known but not fully understood [6] . A major regulator of cell cycle progression in mammalian cells is the RB pathway. RB and its family members, p107 and p130, are best known for their ability to restrict the G1/S transition of the cell cycle, in part through their ability to bind and repress the E2F family of transcription factors. During cell cycle progression, RB family proteins are inactivated by phosphorylation by Cyclin D/CDK4/6 and Cyclin E,A/CDK2 kinases, which are themselves inhibited by INK4a and CIP/KIP family members [7] . RB family proteins also control differentiation, at least in part by their ability to bind multiple lineage-specific transcription factors [7] , [8] , [9] . Furthermore, RB family proteins are found in complexes with chromatin remodelling enzymes, which could help regulate both local and global gene expression [7] . Thus, the RB pathway controls cellular processes that are critically linked to stem cell properties. Accordingly, RB and its two family members p107 and p130 are important regulators of adult stem cell and progenitor populations [10] , [11] , [12] , [13] , [14] , [15] . hESCs are characterized by low expression of D-type Cyclins, and expression and activity of Cyclin E and Cyclin A that differs from the pattern in somatic cells and mouse ESCs (mESCs) [5] . Inhibition of CDK2 or overexpression of its inhibitor p21 CIP1 leads to cell cycle arrest and differentiation in hESCs [16] , [17] , [18] , [19] . But CDK2 key targets in hESCs are still unknown and may involve many factors beyond RB family members [20] , [21] . Interestingly, the CDK2 partner Cyclin A has a different role in the cell cycle of mouse somatic cells and stem cells, including ESCs [22] . Other cell cycle players, CDK6 and CDC25A, functionally interact with self-renewal factors such as Nanog, suggesting that there is a link between the cell cycle and hESC self-renewal [23] . Despite these advances and some known differences between mESCs and hESCs, the role of the cell cycle machinery in hESC pluripotency and self-renewal remains largely unexplored. Here we investigated the role of RB family members in the cell cycle and other aspects of the biology of hESCs. Our results show that hESCs have a specific requirement for the RB family in cell cycle progression, cell survival and their long-term self-renewal. RB activation in hESCs induces cell cycle arrest and death During cell cycle progression, hypophosphorylated RB molecules are able to inhibit S-phase entry. Both hypo- and hyperphosphorylated RB is present in actively dividing hESCs ( Fig. 1a ) and small amounts of RB can be immunoprecipitated with E2F1 from hESC extracts, suggesting there is a small pool of active RB in hESCs ( Fig. 1b ). To investigate RB’s role in hESCs, we constructed a doxycycline-inducible lentiviral vector to ectopically express HA-tagged RB ( Supplementary Fig. S1a ). Expression of HA-RB led to no difference in the formation of colonies positive for alkaline phosphatase (AP) activity, a characteristic of undifferentiated hESCs ( Fig. 1c ). Similarly, expression of an RB-GFP fusion by transient transfection did not significantly change the proliferation of hESCs compared with a GFP control. In contrast, transient expression of a constitutively active (non-phosphorylatable) form of RB (RB7LP-GFP) [24] led to a significant decrease in proliferation ( Fig. 1d ), suggesting that high CDK activity rapidly inactivates most of the RB pool in hESCs. Similar observations were made in mESCs ( Supplementary Fig. S1b ). 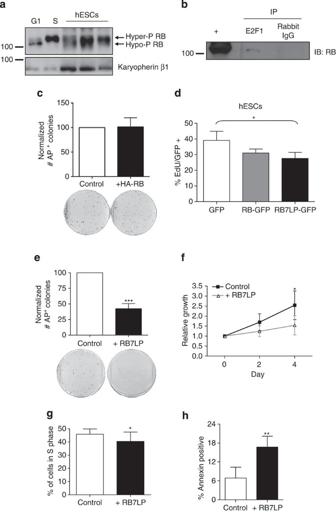Figure 1: Activation of RB in hESCs leads to cell cycle arrest and cell death. (a) Immunoblot analysis detects hyper- and hypo-phosphorylated forms of RB protein in three independent hESC lines. (b) RB co-immunoprecipitates with E2F1, but not control IgG, in hESCs. Input is shown on the left (+). (c) Quantification of stably infected control and HA-RB-expressing hESC colonies growing from single cells and positive for AP activity. Representative pictures shown below. (d) Quantification of EdU-positive cells out of all GFP-positive hESCs transiently transfected with either GFP, RB-GFP or RB7LP-GFP (*,P<0.05;n=3). (e) Quantification of stably infected control and RB7LP-GFP-expressing hESC colonies growing from single cells and positive for AP activity. Representative pictures shown below. (***,P<0.0001;n=5). (f) MTT assay of stably infected control and RB7LP-GFP-expressing hESCs (*,P<0.05;n=4). (g) FACS analysis (S phase) of stably infected control hESCs and hESCs expressing of RB7LP-GFP (*,P<0.05,n=4). (h) Analysis of apoptotic cell death measured by Annexin V staining in control and mutant hESCs (**,P<0.01;n=4). Data are represented as mean±s.d. Molecular weight (in kDa) is shown on the left side of the immunoblots. Figure 1: Activation of RB in hESCs leads to cell cycle arrest and cell death. ( a ) Immunoblot analysis detects hyper- and hypo-phosphorylated forms of RB protein in three independent hESC lines. ( b ) RB co-immunoprecipitates with E2F1, but not control IgG, in hESCs. Input is shown on the left (+). ( c ) Quantification of stably infected control and HA-RB-expressing hESC colonies growing from single cells and positive for AP activity. Representative pictures shown below. ( d ) Quantification of EdU-positive cells out of all GFP-positive hESCs transiently transfected with either GFP, RB-GFP or RB7LP-GFP (*, P <0.05; n =3). ( e ) Quantification of stably infected control and RB7LP-GFP-expressing hESC colonies growing from single cells and positive for AP activity. Representative pictures shown below. (***, P <0.0001; n =5). ( f ) MTT assay of stably infected control and RB7LP-GFP-expressing hESCs (*, P <0.05; n =4). ( g ) FACS analysis (S phase) of stably infected control hESCs and hESCs expressing of RB7LP-GFP (*, P <0.05, n =4). ( h ) Analysis of apoptotic cell death measured by Annexin V staining in control and mutant hESCs (**, P <0.01; n =4). Data are represented as mean±s.d. Molecular weight (in kDa) is shown on the left side of the immunoblots. Full size image To further investigate RB function in hESCs, we stably infected hESCs with a lentiviral vector expressing RB7LP-GFP upon doxycycline administration ( Supplementary Fig. S1c ). Induction of RB7LP-GFP led to a diminished ability to form AP-positive colonies ( Fig. 1e ) and to the presence of small AP-negative colonies, suggesting that overexpression of active RB can result in loss of some stem cell features ( Supplementary Fig. S1d ). RB7LP-GFP expression also led to a decrease in population growth ( Fig. 1f ) and in the number of hESCs progressing through S phase ( Fig. 1g ), and increased cell death ( Fig. 1h and Supplementary Fig. S1e ). Immunoblot analysis showed no significant changes in the phosphorylation of CDK substrates upon RB7LP expression ( Supplementary Fig. S1f ), suggesting that overexpression of the mutant RB7LP protein did not act as a dominant negative form of RB that may titer CDK activity. These experiments indicate that expression of active RB in hESCs leads to a small decrease in proliferation, increased differentiation, and increased cell death. Activation of p53 follows RB activation in hESCs A microarray analysis showed that RB activation in hESCs is associated with a significant decrease in expression of genes implicated in DNA replication and cell cycle ( Supplementary Fig. S1g , Supplementary Table S1 ). Analysis of regulatory elements potentially controlling the expression of these downregulated genes using Distant regulatory elements of co-regulated genes (DiRE) [25] showed an enrichment for E2F targets ( Supplementary Fig. S1h , bottom). The transcription factor tool WebGestalt [26] also found an enrichment for E2F targets in genes downregulated upon RB activation. When we specifically examined E2F target genes [27] that were significantly deregulated ( P <0.05) in our microarray data, we found that the vast majority of E2F targets had decreased expression level in hESCs with RB activation compared with controls ( Fig. 2a ). Protein levels of the E2F target and RB family member p107 also decreased upon RB7LP-GFP expression, whereas p130, which is not an E2F target, remained unchanged ( Fig. 2b ). RB activation in hESCs was also associated with a significant increase in the expression of markers of embryonic development and cellular differentiation, including primitive differentiation markers, such as GATA4 , GATA6 , as well as other differentiation markers, including EOMES , NEFL and MIXL1 ( Supplementary Table S1 , Fig. 2c and data not shown). At this early time point, expression of the pluripotency genes OCT4 and NANOG remained unchanged ( Fig. 2c ). Treatment of hESCs with the E2F inhibitor HLM006474 (ref. 28 ) significantly decreased hESC proliferation ( Fig. 2d ) and led to an increase in cell death ( Fig. 2e ) and in differentiation markers (data not shown). This similarity between the phenotypes of RB overexpression and E2F inhibition suggests that the main mechanism of RB action in the regulation of cell cycle progression in hESCs is inhibition of E2F activity, similar to what has been observed in other cell types. 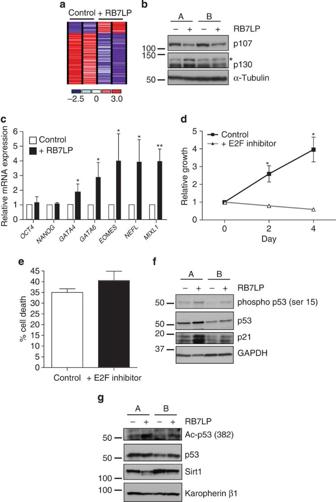Figure 2: Increased differentiation and decreased E2F activity reduce hESC self-renewal upon RB activation. (a) E2F target genes that were significantly differentially regulated (P<0.05) between control hESCs and those with RB overexpression. (b) Immunoblot analysis of p107 and p130 levels upon RB7LP expression. * marks a non-specific band. A and B indicate two independent hESC infections. Tubulin serves as a loading control. (c) RT–qPCR analysis of the expression levels of markers of differentiation in control and mutant hESCs (*,P<0.05; **,P<0.01,n=4, except Nanogn=2). (d) MTT assay of control (DMSO treated) and E2F inhibitor-treated hESCs (*,P<0.05,n=3). (e) Analysis of cell death measured by Annexin V/PI staining in control (DMSO treated) and E2F inhibitor-treated hESCs (n=3). (f) Immunoblot analysis of phospho-p53, p53 and p21 levels upon RB activation in hESCs. A and B indicate two independent hESC infections. GAPDH serves as a loading control. (g) Immunoblot analysis of acetyl-p53, p53 and Sirt1 levels upon expression of RB7LP in hESCs. A and B indicate two independent hESC infections. Karyopherin serves as a loading control. Data are represented as mean±s.d. Molecular weight (in kDa) is shown on the left side of the immunoblots. Figure 2: Increased differentiation and decreased E2F activity reduce hESC self-renewal upon RB activation. ( a ) E2F target genes that were significantly differentially regulated ( P <0.05) between control hESCs and those with RB overexpression. ( b ) Immunoblot analysis of p107 and p130 levels upon RB7LP expression. * marks a non-specific band. A and B indicate two independent hESC infections. Tubulin serves as a loading control. ( c ) RT–qPCR analysis of the expression levels of markers of differentiation in control and mutant hESCs (*, P <0.05; **, P <0.01, n =4, except Nanog n =2). ( d ) MTT assay of control (DMSO treated) and E2F inhibitor-treated hESCs (*, P <0.05, n =3). ( e ) Analysis of cell death measured by Annexin V/PI staining in control (DMSO treated) and E2F inhibitor-treated hESCs ( n =3). ( f ) Immunoblot analysis of phospho-p53, p53 and p21 levels upon RB activation in hESCs. A and B indicate two independent hESC infections. GAPDH serves as a loading control. ( g ) Immunoblot analysis of acetyl-p53, p53 and Sirt1 levels upon expression of RB7LP in hESCs. A and B indicate two independent hESC infections. Karyopherin serves as a loading control. Data are represented as mean±s.d. Molecular weight (in kDa) is shown on the left side of the immunoblots. Full size image Binding sites for transcription factors involved in differentiation, such as SMAD and E47, and cell death, such as p53, were also identified in the regulatory regions of genes whose expression was upregulated by active RB ( Supplementary Fig. S1h , top). Gene set enrichment analysis (GSEA) identified a decrease in categories representing cell cycle, DNA polymerase and various types of metabolism in RB7LP-expressing hESCs, while revealing significant enrichments in p53 signalling, cell communication and apoptosis ( Supplementary Table S2 ). We observed a slight stabilization of p53 and increased expression of its target p21 upon RB activation ( Fig. 2f ), without visible DNA damage ( Supplementary Fig. S1i ). Loss of activating E2F activity in mouse retinal progenitors decreases expression of Sirt1 , an E2F target gene and a p53 deacetylase, leading to increased p53 activity and apoptosis [29] . We observed a similar decrease in Sirt1 as well as a concomitant increase in p53 acetylation at lysine 382 in hESCs with active RB, suggesting that a similar mechanism exists in hESCs for activating p53 upon decreased E2F activity ( Fig. 2g ). Collectively, these experiments indicate that increased RB activity in exponentially growing hESC populations results in a decrease in self-renewal through decreased proliferation combined with differentiation and cell death through inhibition of E2F and activation of p53. RB family inactivation in hESCs blocks their expansion To investigate the effects of loss of RB function in hESCs, we constructed inducible lentiviral vectors expressing short hairpin RNA (shRNA) molecules against human RB ( shRB ). Addition of doxycycline to the culture medium specifically decreased RB protein levels ( Supplementary Fig. S2a ) but did not affect cell cycle or self-renewal ( Supplementary Fig. S2b,c ). Thus, while a pool of RB molecules is active in hESCs ( Fig. 1 ), decreasing RB levels is not sufficient to change the biology of hESCs in these assays. RB, p107 and p130 are expressed in several hESCs lines [30] ( Fig. 2a and Supplementary Fig. S2d ). To block potential compensatory mechanisms by p107 or p130 upon RB loss [31] , we generated an inducible lentiviral vector that expresses the dl1137 mutant of SV40 T antigen (T 121 ) ( Supplementary Fig. S3a ). T 121 binds to and functionally inactivates all members of the RB family but not p53 (refs 32 , 33 ). Surprisingly, we found that T 121 expression severely inhibited the growth of hESCs ( Fig. 3a ) and reduced their ability to undergo normal self-renewal and proliferation ( Fig. 3b ). Expression of the K1 mutant form of T 121 , which disrupts binding to the RB family [34] , did not affect the colony-forming ability of hESCs ( Supplementary Fig. S3b–e ). Genetic inactivation of the entire Rb gene family [31] , [35] had no effect on the growth of mESC populations ( Fig. 3d ). Furthermore, T 121 expression in mESCs did not significantly affect their ability to produce undifferentiated colonies ( Fig. 3f and Supplementary Fig. S3f ). hESCs have been shown to have more characteristics in common with mouse EpiSCs (mEpiSCs) than mESCs [36] , raising the possibility that the differences observed in ESCs from the two species may represent a different requirement for the RB family at different developmental stages (see Discussion). Nevertheless, these experiments indicate that RB family function is required for the expansion of hESC populations. 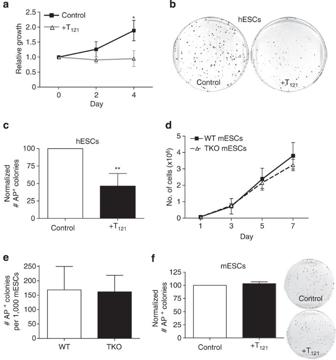Figure 3: Functional inactivation of the RB family alters hESC proliferation. (a) MTT assay of control and T121-expressing hESCs (*,P<0.05;n=6). (b) Representative photographs of control and T121-expressing hESC colonies growing from single cells and positive for AP activity. (c) Quantification of panelb(**,P<0.01;n=5). (d) Wild-type (WT) and TKO mESCs were plated at equal density and then counted every other day (WTn=3; TKOn=5). (e) WT and TKO mESCs produced a similar number of AP+colonies when plated at low density (n=5). (f) Quantification of the number of AP+colonies following T121expression in mESCs. Representative plates of control and T121-expressing mESCs are shown below. Data are represented as mean±s.d. Figure 3: Functional inactivation of the RB family alters hESC proliferation. ( a ) MTT assay of control and T 121 -expressing hESCs (*, P <0.05; n =6). ( b ) Representative photographs of control and T 121 -expressing hESC colonies growing from single cells and positive for AP activity. ( c ) Quantification of panel b (**, P <0.01; n =5). ( d ) Wild-type (WT) and TKO mESCs were plated at equal density and then counted every other day (WT n =3; TKO n =5). ( e ) WT and TKO mESCs produced a similar number of AP + colonies when plated at low density ( n =5). ( f ) Quantification of the number of AP + colonies following T 121 expression in mESCs. Representative plates of control and T 121 -expressing mESCs are shown below. Data are represented as mean±s.d. Full size image RB family mutant hESCs display increased cell death To determine how the loss of RB family function leads to a defect in self-renewal and proliferation of hESCs, we first assessed pluripotency and early differentiation markers. Expression of the pluripotency genes OCT4 and NANOG and of the early embryonic differentiation markers GATA4 and GATA6 was not significantly altered after 4 days of T 121 expression ( Fig. 4a ), suggesting that spontaneous differentiation was not responsible for the observed decrease in the ability to form undifferentiated colonies. In contrast, we found that the percentage of dead cells was significantly increased following T 121 expression compared with controls ( Fig. 4b ). T 121 -expressing hESCs also displayed a significant increase in the percentage of cells in the G2/M phase of the cell cycle after induction of T 121 ( Fig. 4c ). This defect was not observed in cells expressing the K1 mutant form of T 121 ( Supplementary Fig. S3g,h ). Using a protocol to direct the general differentiation of hESCs, we found that hESCs expressing T 121 had a decreased or delayed ability to differentiate, as assessed by expression of markers for each of the germ layers after 2 weeks of differentiation ( Fig. 4e ). To better understand the molecular basis for the phenotypes observed, we examined global gene expression profiles in control hESCs and hESCs expressing T 121 for 3 days by microarray analysis. Fewer than 300 genes were significantly differentially expressed between the two groups ( P <0.05) ( Supplementary Fig. S4a–c ). Among the list of genes significantly upregulated in hESCs expressing T 121 , the top categories were related to cell death ( Supplementary Fig. S4b ). There were very few genes significantly downregulated in T 121 -expressing cells, but GSEA revealed a decrease in various amino-acid metabolism pathways along with lipid and steroid biosynthetic pathways, which is consistent with a decreased need for these molecules during cell cycle arrest ( Supplementary Table S3 ). Thus, inactivation of the RB family by T 121 increases cell death and promotes a G2/M arrest in hESC populations, inhibiting both long-term growth and differentiation. 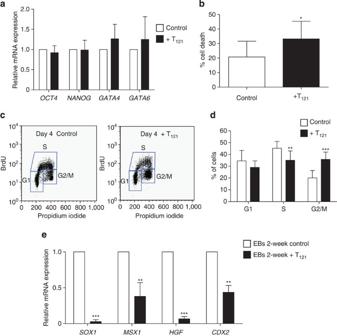Figure 4: Inhibition of RB family function results in increased cell death and cell cycle arrest in hESCs. (a) RT–qPCR analysis of markers of pluripotency and early differentiation in control and T121-expressing hESCs (n=6). (b) Analysis of apoptotic cell death measured by Annexin V/PI staining in control and mutant hESCs (*,P<0.05;n=6). (c) Representative FACS analysis of the cell cycle profiles of control hESCs and hESCs expressing of T121. (d) Quantification of panelc(**,P<0.01; ***,P<0.0001;n=7). (e) RT–qPCR analysis of markers of the three germ layers after 2 weeks of differentiation including ectoderm (SOX1), mesoderm (MSX1), endoderm (HGF) and trophoblast (CDX2) lineages (**,P<0.01; ***,P<0.0001;n≥4). Data are represented as mean±s.d. Figure 4: Inhibition of RB family function results in increased cell death and cell cycle arrest in hESCs. ( a ) RT–qPCR analysis of markers of pluripotency and early differentiation in control and T 121 -expressing hESCs ( n =6). ( b ) Analysis of apoptotic cell death measured by Annexin V/PI staining in control and mutant hESCs (*, P <0.05; n =6). ( c ) Representative FACS analysis of the cell cycle profiles of control hESCs and hESCs expressing of T 121 . ( d ) Quantification of panel c (**, P <0.01; ***, P <0.0001; n =7). ( e ) RT–qPCR analysis of markers of the three germ layers after 2 weeks of differentiation including ectoderm ( SOX1 ), mesoderm ( MSX1 ), endoderm ( HGF ) and trophoblast ( CDX2 ) lineages (**, P <0.01; ***, P <0.0001; n ≥4). Data are represented as mean±s.d. Full size image Activation of E2F and p53 programs RB family mutant hESCs We noted the absence of groups of genes regulated by E2F in the bioinformatics analysis from T 121 -expressing hESCs compared with their controls. Indeed, the expression of several classical E2F target genes, including p107 , Cyclin A2 , Cyclin E1 and E2F1 itself was unchanged in hESCs upon expression of T 121 by RT–qPCR analysis ( Fig. 5a ). In contrast, these same E2F targets genes were significantly upregulated in human fibroblasts expressing T 121 ( Fig. 5b ). However, a subset of E2F targets involved in apoptosis was upregulated in hESCs expressing T 121 in the microarray analysis ( DDB2 , GADD45g and Tp53INP1 ) and by RT–qPCR analysis ( Caspase 3 and Caspase 8 ) ( Fig. 5c ). These cell death genes were not upregulated by T 121 in human fibroblasts ( Fig. 5d ). These results indicate that hESCs are still responsive to the upregulation of E2F activity induced by loss of RB family function. However, only a very specific subset of E2F targets is induced by T 121 in hESCs. These cell death genes seem to be sensitive to increased E2F activity specifically in hESCs rather than fibroblasts, providing one possible explanation for the death observed in T 121 -expressing hESCs. 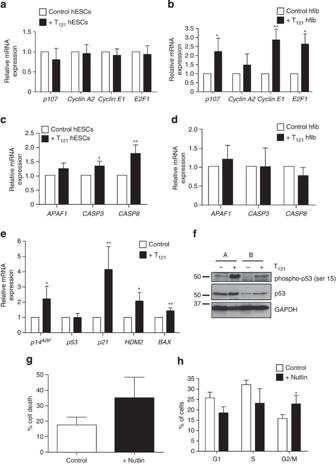Figure 5: A subset of E2F target genes involved in cell death is upregulated in hESCs expressing T121. RT–qPCR analysis of classical cell cycle genes and E2F targets in control and T121-expressing hESCs (a,n≥3) and human fibroblasts (hfib) (b, *,P<0.05; **,P<0.01;n=4). RT–qPCR analysis of cell death genes and E2F targets in control and T121-expressing hESCs (c, *,P<0.05; **,P<0.01;n=5) and human fibroblasts (d,n=4). (e) RT–qPCR analysis of p53 target genes in control hESCs and hESCs expressing T121(*,P<0.05; **,P<0.01;n=5). (f) Immunoblot analysis of p53 and phospho-p53 expression in hESCs with (+) or without (−) T121. A and B indicate two independent hESC infections. (g) Analysis of apoptotic cell death measured by Annexin V/PI staining in control hESCs (DMSO treated) and nutlin-treated hESCs (n=3). (h) BrdU/PI FACS analysis of the cell cycle of controls and hESCs treated with 10 μM nutlin for 2 days (*P<0.05;n=3). Data are represented as mean±s.d. Molecular weight (in kDa) is shown on the left side of the immunoblots. Figure 5: A subset of E2F target genes involved in cell death is upregulated in hESCs expressing T 121 . RT–qPCR analysis of classical cell cycle genes and E2F targets in control and T 121 -expressing hESCs ( a , n ≥3) and human fibroblasts (hfib) ( b , *, P <0.05; **, P <0.01; n =4). RT–qPCR analysis of cell death genes and E2F targets in control and T 121 -expressing hESCs ( c , *, P <0.05; **, P <0.01; n =5) and human fibroblasts ( d , n =4). ( e ) RT–qPCR analysis of p53 target genes in control hESCs and hESCs expressing T 121 (*, P <0.05; **, P <0.01; n =5). ( f ) Immunoblot analysis of p53 and phospho-p53 expression in hESCs with (+) or without (−) T 121 . A and B indicate two independent hESC infections. ( g ) Analysis of apoptotic cell death measured by Annexin V/PI staining in control hESCs (DMSO treated) and nutlin-treated hESCs ( n =3). ( h ) BrdU/PI FACS analysis of the cell cycle of controls and hESCs treated with 10 μM nutlin for 2 days (* P <0.05; n =3). Data are represented as mean±s.d. Molecular weight (in kDa) is shown on the left side of the immunoblots. Full size image We found that another E2F target gene related to apoptosis, p14 ARF , which encodes a p53 activator, was induced by expression of T 121 in hESCs ( Fig. 5e ), together with, several p53 target genes involved in apoptosis (for example, PHLDA3, TNF10b ), including genes that are both p53 and E2F targets (for example, DDB2, Tp53INP1 ). Furthermore, the canonical p53 target genes CDKN1A (coding for p21 CIP1 ), HDM2 and BAX , were all induced in T 121 -expressing hESCs, whereas p53 mRNA levels remained unchanged ( Fig. 5e ). These E2F and p53 targets genes were unchanged in Rb family triple knockout (TKO) mESCs compared with wild-type mESCs ( Supplementary Fig. S4d,e ). Finally, p53 protein levels, as well as p53 phosphorylation at serine 15, was increased in hESCs expressing T 121 compared with control ( Fig. 5f ), whereas p53 and p21 remained unchanged in T 121 K1 mutant expressing hESCs ( Supplementary Fig. S4f ), further indicating that the p53 pathway was activated in hESCs upon decreased activity of the RB family. However, this activation of p53 seems to be occurring independently of an increase in DNA damage ( Supplementary Fig. S4g–i ). Inhibition of p53-p21 module rescues mutant phenotypes We next tested the possibiity that p53 could be responsible for the increased cell death and cell cycle arrest observed in T 121 -expressing hESCs. We found that treatment of hESCs with the HDM2 inhibitor nutlin activated p53 ( Supplementary Fig. S5a ), increased cell death ( Fig. 5g ), and led to a decrease in self-renewal and a cell cycle arrest in G2/M in hESCs ( Supplementary Fig. S5b and Fig. 5h ). To test whether p53 activity was necessary to produce the G2 arrest caused by T 121 in hESCs, we knocked down p53 in these cells ( shp53 ) ( Supplementary Fig. S5c ). Activation of p53 and p21 by T 121 was reduced, although not completely abrogated by the shp53 molecules, whereas HDM2 , BAX and PUMA activation was rescued by p53 knockdown ( Fig. 6a and Supplementary Fig. S5d ). Knockdown of p53 partly rescued the decrease in the ability of hESCs expressing T 121 to form AP-positive colonies ( Fig. 6b ). hESCs expressing shp53 and T 121 still arrested in the G2/M phase ( Fig. 6c ) but displayed reduced apoptosis compared with hESCs expressing T 121 with the control shRNA targeting GFP ( Supplementary Fig. S5e ). 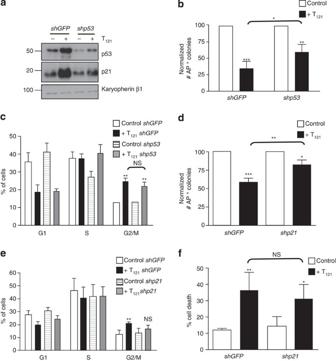Figure 6: Rescue of cell cycle phenotypes in T121-expressing hESCs through knockdown of the p53-p21 module. (a) Immunoblot analysis of p53 and p21 expression in hESCs with (+) or without (−) T121also expressing shRNAs against eitherGFPorp53. (b) Quantification of the number of AP+colonies followingp53knockdown in T121-expressing and control hESCs. (*,P<0.05; **,P<0.01; ***,P<0.001;n=3). (c) Quantification of cell cycle profiles by FACS analysis in hESC populations with or without T121and with or withoutp53knockdown (**,P<0.01;n=2). NS indicates a non-significant difference. (d) Quantification of the number of AP+colonies followingp21knockdown in T121-expressing and control hESCs (*,P<0.05; **P<0.01; ***,P<0.001;n=4). (e) Quantification of cell cycle profiles by FACS analysis in hESC populations with or without T121and with or withoutp21knockdown **,P<0.01;n=4) (f) Analysis of apoptotic cell death measured by Annexin V/PI staining in control andshp21hESCs with or without expression of T121(*,P<0.05; **,P<0.01;n=4). Data are represented as mean±s.d. Molecular weight (in kDa) is shown on the left side of the immunoblots. Figure 6: Rescue of cell cycle phenotypes in T 121 -expressing hESCs through knockdown of the p53-p21 module. ( a ) Immunoblot analysis of p53 and p21 expression in hESCs with (+) or without (−) T 121 also expressing shRNAs against either GFP or p53 . ( b ) Quantification of the number of AP + colonies following p53 knockdown in T 121 -expressing and control hESCs. (*, P <0.05; **, P <0.01; ***, P <0.001; n =3). ( c ) Quantification of cell cycle profiles by FACS analysis in hESC populations with or without T 121 and with or without p53 knockdown (**, P <0.01; n =2). NS indicates a non-significant difference. ( d ) Quantification of the number of AP + colonies following p21 knockdown in T 121 -expressing and control hESCs (*, P <0.05; ** P <0.01; ***, P <0.001; n =4). ( e ) Quantification of cell cycle profiles by FACS analysis in hESC populations with or without T 121 and with or without p21 knockdown **, P <0.01; n =4) ( f ) Analysis of apoptotic cell death measured by Annexin V/PI staining in control and shp21 hESCs with or without expression of T 121 (*, P <0.05; **, P <0.01; n =4). Data are represented as mean±s.d. Molecular weight (in kDa) is shown on the left side of the immunoblots. Full size image We observed that p21, but none of the other canonical p53 targets, was still induced in hESCs expressing T 121 with knockdown of p53 as compared with the control ( Supplementary Fig. S5d ). p21 is regulated in both p53-dependent and -independent manners, including by E2F [37] . We explored whether activation of p21 was a critical factor in the phenotypes displayed in hESCs expressing T 121 . Knockdown of p21 in hESCs ( Supplementary Fig. S5f ) resulted in a significant rescue in the colony-forming ability of hESCs expressing T 121 ( Fig. 6d ). Furthermore, shp21 hESCs expressing T 121 showed a significant rescue of the G2/M arrest seen in control T 121 -expressing cells ( Fig. 6e ). However, knockdown of p21 did not rescue the increased cell death or the differentiation defect induced by T 121 ( Fig. 6f and Supplementary Fig. S5g ). Together, these results indicate that activation of p21 upon functional RB family loss in hESCs has a key role in reducing colony-forming ability and arresting these cells in G2/M, whereas p53 activation has a substantial role in inducing cell death. Genomic instability is increased in hESCs expressing T 121 Recent work has pointed to RB as a critical regulator of genomic stability (reviewed in ref. 38 ). We found that hESCs expressing T 121 for 6 days had an increase in the percentage of >4 N cells compared with controls ( Fig. 7a ). The absence of a defined 8 N peak suggested that T 121 -expressing hESCs were not simply tetraploid but may instead carry a variety of genomic changes. Because of the G2 arrest that results from loss of RB family function, we were unable to obtain many metaphase spreads from hESCs expressing T 121 . To overcome this limitation, we devised a scheme to ‘pulse’ the cells with RB family loss for 3 days and then allow the cells to recover for a similar number of days. This pulse was repeated twice before karyotype analysis ( Fig. 7c ). Using this assay, we found that hESCs pulsed with T 121 expression (T 121 on/off) had fewer normal karyotypes than the controls ( Supplementary Fig. S6a ). Independent preparations of metaphase spreads among multiple hES cell lines analysed by spectral karyotyping (SKY) revealed a significant increase in chromosomal gains among hESCs expressing T 121 on/off ( Fig. 7d ). Chromosomal gains and losses were the primary genomic changes, although a few translocations were also observed in hESCs expressing T 121 , as well as a few whole genome duplications ( Supplementary Fig. S6b ). These results show that the presence of functional RB family is essential in hESCs to maintain genomic stability, further indicating that the activity of the RB family must be tightly controlled to enable the expansion of functional hESCs. Furthermore, we observed that knockdown of p21 did not rescue the genomic instability seen upon loss of RB family function in hESCs ( Fig. 7f ). Accordingly, we found fewer normal karyotypes (40 chromosomes) of Rb family TKO mESCs, which do not display any cell cycle effects like those seen in hESCs, compared with controls ( Fig. 7g ). Collectively, these results suggest an essential role for the RB family in maintaining genomic stability in human and mouse ESCs, independent from its role in the cell cycle. 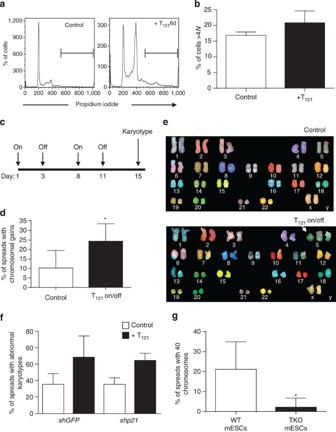Figure 7: ES cells display genomic instability upon loss of RB family function. (a) Representative PI FACS analysis of control hESCs and hESCs expressing T121for 6 days. (b) Quantification of panela(n=3). (c) hESCs were pulsed with T121expression twice for 3 days each before analysis of metaphase spreads. (d) Quantification of the number of spreads with chromosome gains in control hESCs and hESCs expressing T121grown following the protocol in panelc(*,P<0.05;n=3). A total of 75 metaphase spreads were analysed by SKY for the controls and 85 for T121on/off. (e) Example of a normal control and a chromosomal gain from the analysis in paneld. Note the extra chromosome 5 is the mutant hESC spread. (f) Analysis of metaphase spreads in control orshp21hESCs pulsed with T121two times or cultured alongside (n=3). Approximately 10–20 spreads were counted for each condition and experimental replicate. (g) Analysis of metaphase spreads in control orRbfamily TKO mESCs (*,P<0.05;n=5). Approximately 10 spreads were counted for each cell line. Data are represented as mean±s.d. Figure 7: ES cells display genomic instability upon loss of RB family function. ( a ) Representative PI FACS analysis of control hESCs and hESCs expressing T 121 for 6 days. ( b ) Quantification of panel a ( n =3). ( c ) hESCs were pulsed with T 121 expression twice for 3 days each before analysis of metaphase spreads. ( d ) Quantification of the number of spreads with chromosome gains in control hESCs and hESCs expressing T 121 grown following the protocol in panel c (*, P <0.05; n =3). A total of 75 metaphase spreads were analysed by SKY for the controls and 85 for T 121 on/off. ( e ) Example of a normal control and a chromosomal gain from the analysis in panel d . Note the extra chromosome 5 is the mutant hESC spread. ( f ) Analysis of metaphase spreads in control or shp21 hESCs pulsed with T 121 two times or cultured alongside ( n =3). Approximately 10–20 spreads were counted for each condition and experimental replicate. ( g ) Analysis of metaphase spreads in control or Rb family TKO mESCs (*, P <0.05; n =5). Approximately 10 spreads were counted for each cell line. Data are represented as mean±s.d. Full size image Here, we present data showing that both too much and too little RB activity is detrimental to self-renewing hESCs. Upregulation of specific E2F targets in hESCs upon functional knockdown of the RB family may have an important role in regulating apoptosis through the p53 pathway and induction of caspases. The cell cycle inhibitor p21 is regulated in both p53-dependent and independent manners to arrest hESCs upon loss of RB family function. Based on these observations, we propose a model where RB family activity is critical to maintain the balance between proliferation and cell survival in hESCs ( Fig. 8 ). 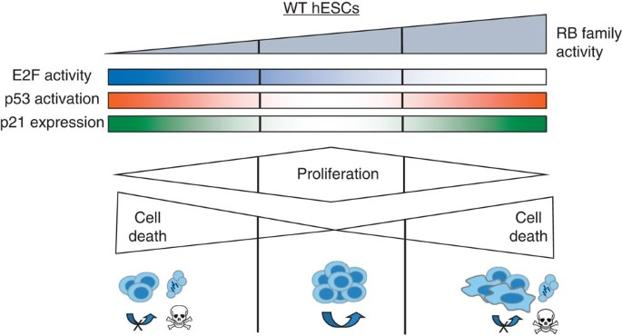Figure 8: Model of RB action in human embryonic stem cells. When RB is activated, E2F transcription factors are inhibited and hESCs exit the cell cycle and undergo cell death and differentiation. When the RB family is inactivated in hESCs, increased E2F activity triggers apoptosis through p53-dependent and independent pathways in addition to cell cycle arrest through induction of p21. These cell cycle regulatory networks are specific to human ES cells when compared with mouse ES cells. Figure 8: Model of RB action in human embryonic stem cells. When RB is activated, E2F transcription factors are inhibited and hESCs exit the cell cycle and undergo cell death and differentiation. When the RB family is inactivated in hESCs, increased E2F activity triggers apoptosis through p53-dependent and independent pathways in addition to cell cycle arrest through induction of p21. These cell cycle regulatory networks are specific to human ES cells when compared with mouse ES cells. Full size image Inactivation of the three RB family proteins does not affect the proliferation of mESCs (refs 31 , 35 and this study) but it results in G2 arrest and cell death in hESCs. mESCs and hESCs are known to display a number of significant differences [5] . For instance, hESCs cycle more slowly [39] and RB molecules are less hyperphosphorylated in hESCs than in mESCs [40] . Thus, it is tempting to speculate that mESCs have adapted to the complete loss of function of RB family members, whereas inactivation of the RB family in hESCs can still acutely result in the activation of specific E2F targets, including genes involved in cell death. Alternatively, hESCs are more similar to mouse EpiSCs and most likely represent a later stage of development than mESCs [36] . For example, both mEpiSCs and hESCs are dependent on FGF signalling, display poor survival of single cells and have a longer cell cycle and different morphology compared with mESCs [36] , [41] . However, hESCs and mEpiSCs do have some molecular differences, including the role of FGF signalling [42] . We have begun to investigate the consequences of inactivating the RB pathway in mouse epiblast cells by generating Rb family triple knockout ‘induced EpiSCs’ [43] from Rb family conditional knockout mouse embryonic fibroblasts (MEFs) and found no detrimental consequences upon loss of Rb family function in this cell type ( Supplementary Fig. S7a–f ). This observation suggests that the phenotypes we observed in hESCs are not due to their specific embryonic origin. More work will need to be done to fully understand the role of the RB family in mEpiSCs and to compare that role to both human and mouse ESCs. Nevertheless, our observations highlight the importance of studying basic signalling networks in hESCs and further add to the emerging body of literature suggesting substantial biological differences between mouse and human ESCs [5] , [39] , [44] , [45] . We found here that overexpression of an active form of RB is sufficient to trigger cell cycle arrest and cell death. Although we cannot rule out some non-physiological effects of using a mutant form of RB, previous studies have shown that RB can be pro-apoptotic in addition to promoting cell cycle arrest [46] . Previous studies have shown that DNA damage and inhibition of CDK4 activity do not activate a G1 checkpoint in hESCs [40] , [47] , [48] . The difference between these studies and ours is probably due to the high CDK2 activity in hESCs, which can inactivate RB family proteins even in the context of low CDK4 activity. Mass spectrometry data have identified CDK2/1 substrates as key mediators of the maintenance of pluripotency [49] and inhibition of CDK2 results in G1 arrest in hESCs [40] . Both activation of RB and inhibition of CDK2 induce the differentiation of arrested hESCs, suggesting that Cyclin/CDK2 complexes and RB family proteins function in the same pathway in hESCs. Constitutive Cyclin E/CDK2 activity in mESCs bypasses the need for MAPK-induced expression of Cyclin D and renders these cells insensitive to differentiation signals that may be mediated by MAPK activity in somatic cells [3] , [50] . These observations identify an RB-p21-CDK2 module as a major regulator of hESC biology and place RB activity at a critical node between proliferation and self-renewal in pluripotent hESCs. A fundamental goal in the RB field is to understand the regulatory networks surrounding the RB pathway that mediate different responses upon the loss of the function of the RB family in various cell types. One potential insight from our work is that basal expression levels of E2F target genes might have a key role in the downstream effects of RB pathway inactivation. For example, Cyclin E is expressed about three times higher in hESCs compared with human fibroblasts ( Supplementary Fig. S7g ). In contrast, both p21 and p14 ARF are expressed at very low levels in hESCs compared with fibroblasts, raising the possibility that any increase in their expression in hESCs may have a larger effect than in fibroblasts ( Supplementary Fig. S7g ). Future work will further elucidate the consequences of changes in the expression of E2F target genes in high- and low-expressing cell types. Our data also indicate that loss of RB family function in mouse and human ESCs results in genomic instability, supporting previous evidence in mESCs [51] . In somatic cells, loss of RB function may result in genomic instability by inducing high levels of MAD2 expression [52] but the levels of MAD2 RNA did not change upon T 121 expression in hESCs ( Supplementary Fig. S6c ). Thus, it is possible that defects in centromeric function and chromosome condensation during mitosis [53] , [54] , [55] are at the root of the genomic instability in RB family mutant ESCs. Our work indicates that the RB family has a key role in maintaining genomic stability in ESCs and a specific role in the proliferation, self-renewal and differentiation of hESCs. RB may therefore functionally connect multiple cellular pathways to ensure the propagation of undifferentiated hESCs and preserve their ability to differentiate. Cell culture hESC lines H9 (Wicell) and LSJ2 (Stanford) were maintained on irradiated feeders as described previously [56] . mTeSR1 (Stem Cell) was used for culturing cells on Matrigel for MTT assay. Lentivirus particles were produced in 293T cells and concentrated using ultracentrifugation. Doxycycline was added to hESCs the day after plating, at a concentration of 1 μg ml −1 except in the case of LSJ2-T 121 hESCs, which were treated with only 40 ng ml −1 to avoid overexpression of the transgene. Two independent infections of H9-T 121 hESCs were analysed. Cells were transfected using Lipofectamine 2000 (Invitrogen) and treated with 2 h of 10 μM of EdU before fixation with 4% paraformaldehyde and staining. A concentration of 10 μM of nutlin was used as described previously [16] . Doxorubicin was added for 8 h at a dose of 0.2 μg ml −1 . Caffeine treatment was 2 mM for 24 h before harvest. The E2F inhibitor HLM0064747 was used at a concentration of 30 μM and was replaced daily. hESCs were directed to differentiate through the formation of embryoid bodies (EBs) using low-attachment plates (E and K Scientific) for 1 week, and then the EBs were plated on gelatin and allowed to differentiate for 1 more week. Media for differentiation was DMEM+20% fetal bovine serum. Generation of iEpiSCs was performed as described previously, using MEF-conditioned media and Rb family conditional TKO (cTKO) MEFS ( Rb lox/lox ; p130 lox/lox ; p107 −/− ) [57] . Low-density plating assay Single-cell suspensions of 10,000 human and 1,000 mouse ESCs were plated on 10 cm plates and cultured for 1 week. Single-cell suspensions of 5,000 iEpiSCs were plated on 6 cm plates and cultured for 1 week. Plates were then stained for AP and the number of positive colonies was counted. Controls were set to 100 in hESCs due to variation among different ESC lines in the efficiency of colony formation from single cells. Vectors for knockdown and overexpression Vectors expressing inducible HA-RB, RB7LP-GFP, T 121 , T 121 K1 and both shRNAs against RB were constructed using the pSLIK vector system [58] pLKO.1 was used to construct vectors containing shRNA against GFP or human p53 . pSicoR [59] was used to construct the vectors containing shRNA against GFP or human p21 . shRNA target sequences are as follows: GFP : 5′-GCAAGCTGACCCTGAAGTTCAT-3′, RB #1: 5′-GGACATGTGAACTTATATA-3′, RB #2: 5′-GAACGATTATCCATTCAAA-3′, p53: 5′-CACCATCCACTACAACTACAT-3′, p21 : 5′-GAATGAGAGGTTCCTAAGA-3′. Cell cycle and cell death assays The analysis of cell cycle profiles was performed on cells incubated 4 h with BrdU and stained with propidium iodide (PI) after fixation, as described [60] . The MTT assay (Invitrogen) was used to analyse cell growth on hESCs plated on Matrigel and cultured in mTeSR for 0, 2 and 4 days of treatment. Quantification of cell death was performed using AnnexinV-FITC and PI or AnnexinV-PE alone according to the manufacturer’s instructions (BD Biosciences). Fluorescence-activated cell sorting (FACS) data were analysed using FlowJo software. RNA and protein analysis Cell pellets were lysed in TRIzol (Invitrogen) DNase-treated using the RNeasy mini kit (Qiagen). Complementary DNA synthesis was performed using the DyNAmo cDNA synthesis kit (Finnzymes) and quantitative PCR was performed using the SYBR GreenER Mastermix (Invitrogen) on an ABI 7900HT Detection System. All samples were run in triplicate and normalized to a TATA-binding protein (TBP) control RT–PCR. The primer sequences used in these experiments are listed in Supplementary Table S4 . Relative quantification was performed to be relative to cells that were not treated with doxycycline. Cell pellets for immunoblotting were prepared as described previously [31] . Membranes were probed with the following antibodies: α-tubulin (Sigma T9026; Sigma), Karyopherin β1 (Santa-Cruz Biotechnology, sc-1919), p21 (Santa-Cruz Biotechnology, sc-397), p53 (Santa-Cruz Biotechnology, sc-126), T121 (Abcam, ab16879-1), RB (Rb4.1; Developmental Studies Hybridoma Bank, University of Iowa), p107 (Santa-Cruz Biotechnology, sc-318), p130 (BD Biosciences, 610621), Kap1 (aka KRIP1, BD Transduction Laboratories, 610680), Phospho-KAP1 (S824, Bethyl Laboratories A300-767A), Phospho-p53 (Ser 15 Cell Signaling 9284), Acetyl-p53 (Human Lys382, Cell Signaling, 2570), Phospho-Histone H2A.X (Ser 139 20E3, Cell Signaling, 9718), Sirt1 (Upstate, 07131), Phospho-(Ser) CDKs Substrate (P-S 2 -100, Cell Signaling, 9477) and GAPDH (Abcam, ab36840). Secondary antibodies conjugated to HRP (Jackson ImmunoResearch) or fluorescent dyes (LI-COR Biosciences) were detected by chemiluminescence or an Odyssey Infrared Imager, respectively. Microarray analysis Total RNA was extracted with TRIzol and hybridized to Human Genome U133 Plus 2.0 arrays (Affymetrix) according to the manufacturer’s instructions. Raw data were analysed with Robust Multichip Average, using quantile normalization, and LIMMA was performed to generate the lists of differentially expressed genes. GO analysis was performed using the WebGestalt Gene Set Analysis Toolkit V2. GSEA was completed on the entire list of differentially expressed genes (Gene Ontology MSigDB databases). DiRE analysis was performed on significant list (FC>1.5 and P -value<0.05) for both up- and downregulated genes in RB7LP and T 121 samples. In this analysis, the Occurrence reflects the number of potential binding sites for specific transcription factors in proximal and distal regulatory regions, whereas the Importance reflects the same numbers relative to the general occurrence of these binding sites in the genome. Primary microarray data are accessible through Gene Expression Omnibus Series accession number GSE29783. Karyotyping Cells for karyotyping or SKY were treated with 10 μl ml −1 KaryoMAX Colcemid Solution (Invitrogen) for 18 h. Warm hypotonic solution (1:1 0.4% potassium chloride and 0.4% sodium citrate) was slowly added to the cells to enhance swelling at 37 °C for 15 min. Carnoy's solution (methanol:glacial acetic acid, 3:1 ratio) was used to fix the cells for 30 min. The cells for karyotyping were dropped onto a pre-cleaned slide and stained with DAPI and metaphase spreads were counted. The cells for SKY were then dropped onto a pre-cleaned slide and hybridized with probes from the SkyPaint DNA kit for human chromosomes (Applied Spectral Imaging) for 2 days in a 37 °C humidified chamber. The stained metaphase spreads were visualized and analysed using the SkyView spectral imaging system (Applied Spectral Imaging). Statistical analysis Two-tailed student t -tests were performed between controls and experimental groups using the software Graphpad Prism. Paired and unpaired t -tests were used where appropriate. One-way ANOVA analysis was used for groups with three or more samples, with Tukey’s post-test for comparisons between groups. J.F.C. performed all the experiments. J.F.C., J.B. and J.S. designed the experiments, analysed the data and wrote the manuscript. How to cite this article: Conklin, J.F. et al. The RB family is required for the self-renewal and survival of human embryonic stem cells. Nat. Commun. 3:1244 doi: 10.1038/ncomms2254 (2012).